A waveguide frequency converter connecting rubidium-based quantum memories to the telecom C-band Coherently converting the frequency and temporal waveform of single and entangled photons will be crucial to interconnect the various elements of future quantum information networks. Of particular importance is the quantum frequency conversion of photons emitted by material systems able to store quantum information, so-called quantum memories. There have been significant efforts to implement quantum frequency conversion using nonlinear crystals, with non-classical light from broadband photon-pair sources and solid-state emitters. However, solid state quantum frequency conversion has not yet been achieved with long-lived optical quantum memories. Here we demonstrate an ultra-low-noise solid state photonic quantum interface suitable for connecting quantum memories based on atomic ensembles to the telecommunication fibre network. The interface is based on an integrated-waveguide nonlinear device. We convert heralded single photons at 780 nm from a rubidium-based quantum memory to the telecommunication wavelength of 1,552 nm, showing significant non-classical correlations between the converted photon and the heralding signal. Photonic quantum memories (QMs) [1] , [2] have been implemented with single atoms and ions [3] , [4] , [5] , [6] , [7] , atomic ensembles [8] , [9] , [10] , [11] , [12] , [13] , [14] and solid state systems [15] , [16] , [17] , [18] . Proofs of principle of short distance elementary quantum networks [19] have been built with these QMs [3] , [4] , [5] , [8] , [20] , [21] , [22] . For long distance implementation of quantum information networks using quantum repeaters [2] , [19] , [23] , [24] , it is required that optical QMs are connected to the optical fibre network. However, despite initial attempts to build QMs operating in the telecom range [25] , [26] , the best current QMs absorb and emit photons in the visible to near infrared range, where losses in optical fibres are significant. To overcome this problem, a possible strategy consists in translating the frequency of the single photons emitted by the QMs to the telecommunication band, in an efficient, noise-free and coherent manner. Quantum frequency conversion (QFC) of photons from rubidium atoms based QMs to 1,367 nm has been demonstrated using four wave mixing in a cold and very dense atomic ensemble [12] , where the input and target wavelengths are fixed by the available atomic transitions. In contrast, QFC in solid state nonlinear materials offers wavelength flexibility and much simpler experimental implementation, as well as prospects for integrated circuits using waveguide configurations [27] , [28] , [29] , [30] , [31] , [32] , [33] , [34] , [35] , [36] , [37] . Frequency down conversion using difference frequency generation (DFG) enables frequency translation from visible to telecom bands and is therefore ideally suited for quantum repeaters applications with emissive QMs [2] . DFG has been demonstrated with single photons from solid state emitters [33] , [35] , [36] and spontaneous parametric down conversion sources [34] , [38] . However, so far QFC using solid state nonlinear devices has not been demonstrated with long-lived optical QMs based on atomic systems. A significant experimental challenge in solid state QFC is to reduce the noise generated by the strong pump beam in the crystal, which is proportional to the input photon duration, to operate in the quantum regime. Now, atomic QMs usually emit photons with durations ranging from tens of nanoseconds [14] , [39] to hundreds of nanoseconds [3] . This is one to three orders of magnitude longer than the photons that have been converted so far from spontaneous parametric down conversion sources [27] , [34] or broad band solid state emitters [33] , [35] , [36] , which typically have subnanosecond durations. This in turn leads to much stronger requirements in terms of noise suppression for the QFC. QFC to telecom wavelength of rubidium resonant coherent light has been recently demonstrated [40] , however, with a level of noise preventing high-fidelity conversion of nonclassical light. In this Article, we demonstrate an ultra-low-noise solid state photonic quantum interface capable of connecting QMs based on atomic ensembles to the telecommunication network. We generate heralded single photons at 780 nm from a cold 87 Rb atomic ensemble QM and convert them to 1,552 nm using DFG in a nonlinear periodically poled lithium niobate (PPLN) waveguide. By combining high QM retrieval efficiency, high QFC efficiency and narrow band filtering, we can operate the combined systems in a regime where a significant amount of non-classical correlations is preserved between the heralding and converted photons. Atomic quantum memory Our experimental setup is shown in Fig. 1 (see also Supplementary Fig. 1 ). It is composed of two main parts, the QM and the QFC device (QFCD). The QM used in this work belongs to the class of the so called ‘emissive’ QMs, where quantum correlations between light and matter are created by a classical laser pulse. It is implemented with an ensemble of laser cooled 87 Rb atoms, following the scheme proposed by Duan et al. [24] (see Methods and Supplementary Note 1 for more details). Single collective spin excitations are created by a 16 ns long weak write pulse at 780 nm, blue detuned by 40 MHz from the | g › to | e › transition (see Fig. 1b ) and heralded by the detection of a photon emitted by spontaneous Raman scattering, called Stokes photon. The collective spin excitation is stored in the atoms for a programmable time (330 ns in our experiment) before being transferred back into a single photon (anti-Stokes) thanks to an 11 ns long read laser pulse resonant with the | s › to | e › transition. The anti-Stokes photon is emitted with high probability in a single spatio-temporal mode thanks to collective interference between all the emitters. It is then coupled with high efficiency (0.7) into a single mode fibre before being detected by a single photon detector (SPD) with efficiency η d,780 =0.43, bypassing the QFCD. 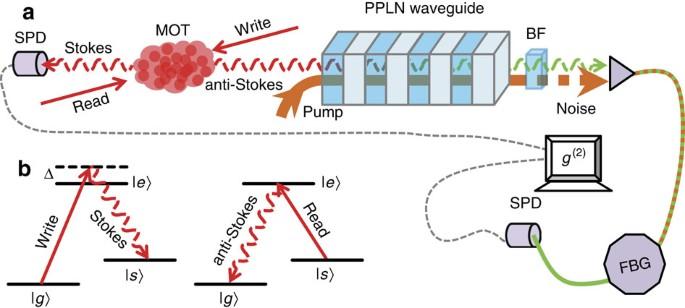Figure 1: Schematic view of the experimental setup. (a) A cold cloud of87Rb atoms confined in a magneto-optical trap (MOT) serves as quantum memory for light. Inelastic scattering of a classical write pulse results in the emission of a Stokes photon, which heralds the presence of a collective spin excitation. A subsequent read pulse maps the atomic state onto an anti-Stokes photon. The retrieved light is sent to a PPLN waveguide, together with a strong pump at 1,569 nm. The 780 nm photons are converted to 1,552 nm by DFG. After conversion, residual pump light is blocked by means of a bandpass filter (BF). The converted light is then coupled in a single mode optical fibre. A fibre Bragg grating filters out the broadband noise generated by the pump. The non-classical nature of the storage, retrieval and conversion processes is probed by measuring the cross-correlation between Stokes and (un)converted anti-Stokes photons. (b) Level scheme used for the DLCZ memory. The write pulse off-resonantly couples the ground state |g› to the excited level |e›. A Stokes photon is emitted with probabilityp, thus creating a single collective excitation to the storage state |s›. During the retrieval process, a pulse resonant with the |s›→|e› transition (read beam) collectively transfers back the atom to the initial state |g› while emitting an anti-Stokes single photon in a well-defined spatio-temporal mode. Figure 1: Schematic view of the experimental setup. ( a ) A cold cloud of 87 Rb atoms confined in a magneto-optical trap (MOT) serves as quantum memory for light. Inelastic scattering of a classical write pulse results in the emission of a Stokes photon, which heralds the presence of a collective spin excitation. A subsequent read pulse maps the atomic state onto an anti-Stokes photon. The retrieved light is sent to a PPLN waveguide, together with a strong pump at 1,569 nm. The 780 nm photons are converted to 1,552 nm by DFG. After conversion, residual pump light is blocked by means of a bandpass filter (BF). The converted light is then coupled in a single mode optical fibre. A fibre Bragg grating filters out the broadband noise generated by the pump. The non-classical nature of the storage, retrieval and conversion processes is probed by measuring the cross-correlation between Stokes and (un)converted anti-Stokes photons. ( b ) Level scheme used for the DLCZ memory. The write pulse off-resonantly couples the ground state | g › to the excited level | e ›. A Stokes photon is emitted with probability p , thus creating a single collective excitation to the storage state | s ›. During the retrieval process, a pulse resonant with the | s ›→| e › transition (read beam) collectively transfers back the atom to the initial state | g › while emitting an anti-Stokes single photon in a well-defined spatio-temporal mode. 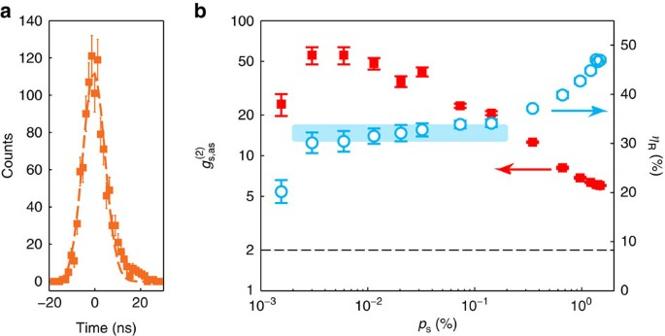Figure 2: Characterization of the DLCZ quantum memory. (a) Temporal shape of anti-Stokes photons. The number of anti-Stokes detection events per time bin (bin size 1.28 ns) conditioned on a Stokes detection over 5 × 106trials is plotted as a function of the arrival time (total integration time 109 s). The data shown correspond tops=0.15%. The dashed line is a Gaussian fit with FWHM=11.4(9) ns. For these data, we haveandηR=35(1)%. (b) Second order cross-correlation function(red plain squares, left axis) and retrieval efficiencyηR(blue empty circles, right axis) as a function of the Stokes detection probabilityps. Forpsbetween 0.002 and 0.2% (shaded area),ηRis constant (32(2)%). Thefunction increases until 56(8), before dropping for lower values ofpsdue to detector dark counts. The dashed line is theclassical limit for two-mode squeezed states. For this plot, the number of trials varies from 4 × 106to 6 × 107. The error bars represent ±1 s.d. assuming Poissonian statistics for the photon counts. Full size image Figure 2a shows the temporal profile of the heralded retrieved anti-Stokes field. We measure a full width at half maximum (FWHM) of 11.4(9)ns, shorter than previous single photons generated by the same method [14] , [39] . We then characterize the non-classical correlations between the Stokes photons and the stored spin excitations. This is realized by measuring the second order cross-correlation function between the Stokes and anti-Stokes fields, defined as g s,as (2) = p s,as /( p s p as ), where p s,as is the probability to detect a coincidence between the two modes and p s ( p as ) is the probability to detect a Stokes (anti-Stokes) photon. p s is proportional to the write pulse intensity. Figure 2b shows a typical measurement of as a function of p s . As expected for this type of source, the degree of correlation increases when decreasing the excitation probability [41] . The measured is well above the classical threshold of 2 for two-mode squeezed states (see Supplementary Notes 1 and 2 ). This suggests that strong non-classical correlations between the Stokes photon and the stored spin excitation are present. Additional measurements demonstrating the non-classical character of the correlations are shown in Supplementary Note 2 (see also Supplementary Fig. 5 ). Also shown in Fig. 2b is the retrieval efficiency η R = p s,as /( p s η d,780 ) corresponding to the probability to find an anti-Stokes photon before the SPD conditioned on the detection of a Stokes photon. In the region where the multi-excitation probability and the Stokes detector dark counts are negligible [41] ( p s between 0.002 and 0.2%), η R is constant and equal to 32(2)% (shaded area on Fig. 2b ). Figure 2: Characterization of the DLCZ quantum memory. ( a ) Temporal shape of anti-Stokes photons. The number of anti-Stokes detection events per time bin (bin size 1.28 ns) conditioned on a Stokes detection over 5 × 10 6 trials is plotted as a function of the arrival time (total integration time 109 s). The data shown correspond to p s =0.15%. The dashed line is a Gaussian fit with FWHM=11.4(9) ns. For these data, we have and η R =35(1)%. ( b ) Second order cross-correlation function (red plain squares, left axis) and retrieval efficiency η R (blue empty circles, right axis) as a function of the Stokes detection probability p s . For p s between 0.002 and 0.2% (shaded area), η R is constant (32(2)%). The function increases until 56(8), before dropping for lower values of p s due to detector dark counts. The dashed line is the classical limit for two-mode squeezed states. For this plot, the number of trials varies from 4 × 10 6 to 6 × 10 7 . The error bars represent ±1 s.d. assuming Poissonian statistics for the photon counts. Full size image Quantum frequency conversion device The heralded anti-Stokes single photon is then directed towards the QFCD where the conversion from 780 nm to 1,552 nm takes place. From the measured η R and the optical transmission between the QM and the QFCD ( η trans =0.77), we infer that, conditioned on a Stokes detection, the number of photons before the QFCD is . The pump light at 1,569 nm and the single photons at 780 nm are combined using a dichroic mirror. Both beams are then coupled into the waveguide where the conversion takes place (see Methods and Supplementary Note 3 ). After conversion, the pump light is blocked by means of two bandpass filters, and the converted light is coupled into a single mode optical fibre. A fibre Bragg grating with a bandwidth of 2.5 GHz and a transmission efficiency of 0.7 then filters out the broadband noise generated in the crystal by the pump beam [40] . The single photons at 1,552 nm are finally detected with an InGaAs avalanche photodiode SPD (detection efficiency η d,1552 =0.1). 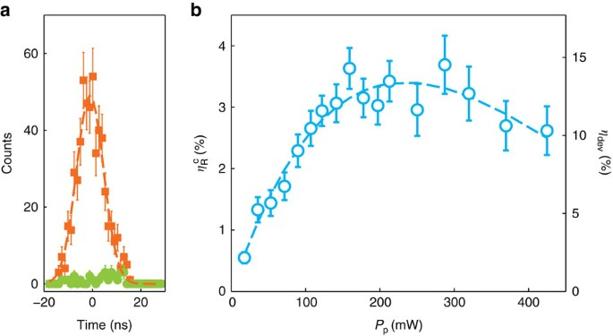Figure 3: Characterization of the quantum frequency conversion device. (a) Converted anti-Stokes photon shape. The conditioned events over 108trials (total integration time 2,180 s) are plotted as orange squares, while the conditioned pump noise is shown as green circles. The measured SNR is 18(5). The time bin size is 1.28 ns. The Stokes detection probability for the measurement isps=0.16% while the pump power isPp=120 mW. For this measurement, we haveand. (b) Conversion efficiency as a function of pump power after the waveguide measured with heralded anti-Stokes photons. The right axis shows the device efficiencyηdevcorresponding to raw conversion efficiency corrected only by the detection efficiency (0.1). The left axis shows, that is, the probability to find a converted photon before the SPD, conditioned on a Stokes detection. The Stokes detection probability for this measurement isps=0.16%. The number of trials varies from 107to 2 × 107. The dashed blue line is a fit of the experimental data using Supplementary equation (3) (seeSupplementary Note 3). The error bars represent ±1 s.d. assuming Poissonian statistics for the photon counts. Figure 3a shows the waveform of the heralded single photons after conversion. The measured temporal profile (FWHM=13(1) ns) is very similar to the input one, which shows that the conversion preserves the waveform of the photons. The noise generated by the pump beam at 1,569 nm is measured by blocking the input of the converter. The measured signal to noise ratio (SNR) of 18(5) gives an upper bound for the value of the cross-correlation function achievable after conversion (see Methods). We also measure the efficiency of the conversion process as a function of the pump power P p measured after the waveguide. Figure 3b shows the device efficiency where is the probability to detect a coincidence after conversion. η dev corresponds to the probability to find a converted photon in a single mode optical fibre after the QFCD (including filtering and fibre coupling) for a single photon input. The data are fitted with the following formula (ref. 32 ). From the fit, we extract η n =120(10)%W −1 cm −2 and η max =13.6(12)%. The maximum achievable device efficiency is limited in our current setup to 17.6% by optical losses, including fibre coupling efficiency (60%) and Bragg grating filter transmission (70%) at the converted wavelength of 1,552 nm, as well as by the waveguide incoupling (60%) and transmission (70%) efficiencies for 780 nm photons. The discrepancy between the measured η max and the theoretical one is attributed to non-perfect mode overlap between the pump and single photon in the waveguide [32] . Figure 3b also displays , which can be considered as the combined efficiency of the QM+QFCD system, including all losses. Figure 3: Characterization of the quantum frequency conversion device. ( a ) Converted anti-Stokes photon shape. The conditioned events over 10 8 trials (total integration time 2,180 s) are plotted as orange squares, while the conditioned pump noise is shown as green circles. The measured SNR is 18(5). The time bin size is 1.28 ns. The Stokes detection probability for the measurement is p s =0.16% while the pump power is P p =120 mW. For this measurement, we have and . ( b ) Conversion efficiency as a function of pump power after the waveguide measured with heralded anti-Stokes photons. The right axis shows the device efficiency η dev corresponding to raw conversion efficiency corrected only by the detection efficiency (0.1). The left axis shows , that is, the probability to find a converted photon before the SPD, conditioned on a Stokes detection. The Stokes detection probability for this measurement is p s =0.16%. The number of trials varies from 10 7 to 2 × 10 7 . The dashed blue line is a fit of the experimental data using Supplementary equation (3) (see Supplementary Note 3 ). The error bars represent ±1 s.d. assuming Poissonian statistics for the photon counts. Full size image Quantum state preservation To verify that the conversion preserves the quantum character of the input light, we measure the second order cross-correlation function after conversion as a function of p s (see Fig. 4 ). As in the case before conversion ( Fig. 2b ), we also observe an increase of non-classical correlations when decreasing the excitation probability, but the maximum is now reached for much higher values of p s because of the background noise induced by the converter pump laser. However, this background is sufficiently low to observe strong non-classical correlations between the heralding photons at 780 nm and the converted photons at 1,552 nm. 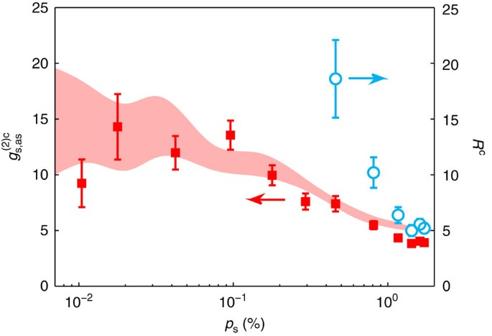Figure 4: Characterization of the quantum memory-quantum frequency converter combined setup. Cross-correlation between Stokes and converted anti-Stokes photons as a function of Stokes detection probability, for a pump power of 140 mW (red plain squares, left axis). The number of trials for this measurement varies from 107to 108. The shaded area represents the expected. It is deduced from the data ofFig. 2bby means of equation (1) (see Methods). The half width represents one s.d. around the mean value. The calculated points have been interpolated with a spline. The measured Cauchy-Schwarz parameterRcis plotted on the right axis (blue empty circles). The unconditional autocorrelation measurement for the converted anti-Stokes field has been measured for a pump power of 120 mW. The error bars represent ±1 s.d. assuming Poissonian statistics for the photon counts. The expected value of the after conversion can be estimated using a simple model taking into account the noise induced by the pump laser, using the following expression (see Methods): Figure 4: Characterization of the quantum memory-quantum frequency converter combined setup. Cross-correlation between Stokes and converted anti-Stokes photons as a function of Stokes detection probability, for a pump power of 140 mW (red plain squares, left axis). The number of trials for this measurement varies from 10 7 to 10 8 . The shaded area represents the expected . It is deduced from the data of Fig. 2b by means of equation (1) (see Methods). The half width represents one s.d. around the mean value. The calculated points have been interpolated with a spline. The measured Cauchy-Schwarz parameter R c is plotted on the right axis (blue empty circles). The unconditional autocorrelation measurement for the converted anti-Stokes field has been measured for a pump power of 120 mW. The error bars represent ±1 s.d. assuming Poissonian statistics for the photon counts. Full size image The shaded area displayed in Fig. 4 corresponds to the expected values taking into account the measured in Fig. 2 and SNR = ·SNR max , where SNR max is the maximal achievable SNR for =1 and can be accurately measured with weak coherent states (see Supplementary Note 3 and Supplementary Fig. 4 ). We find SNR max =85(3). The good agreement between experimental data and expected values suggests that the noise generated from the pump is the only factor degrading the correlations and that further reduction in this noise should lead to even higher non-classical correlations. Finally, to unambiguously prove the non-classical character of the correlations, we also measure the unconditional autocorrelation function for the Stokes ( ) and converted anti-Stokes fields ( ). For classical independent fields, the Cauchy-Schwarz inequality must be satisfied. The values for and are listed in Supplementary Table 1 (see also Supplementary Note 2 ). On the right axis of Fig. 4 , we plot the values of R c measured in our experiment for various p s . The Cauchy-Schwarz inequality is clearly violated, which is a proof of non-classical correlation between Stokes and converted anti-Stokes photons. We now discuss the performances of our QFCD. The measured maximal η dev =13.6(12)% corresponds to an internal waveguide conversion efficiency of 77%. As it is, it would already lead to an increased transmission with respect to the unconverted photon at 780 nm (3 dB km −1 loss) after only ~3 km of fibre (see also Supplementary Fig. 3 ). Further improvement in the device efficiency could be primarily obtained by technical improvements such as decreasing the passive optical losses due to waveguide coupling and transmission, fibre coupling and filtering transmission. For DLCZ type QMs, the quality of the combined QM+QFCD system can be assessed by the measured function [2] . For example, it has been shown that if the DLCZ QM is used to prepare entanglement between Stokes and anti-Stokes photons, the violation of the Clauser-Horne-Shimony-Holt inequality can be calculated as [42] : S ≤2(2) 1/2 . In our experiment, the maximal measured is about 15, which would therefore be sufficient to enable a violation of Bell's inequality if the photons were entangled, for example, in polarization [42] . In that case, the maximal fidelity of the stored and converted qubit would be given by , leading to F c ≤0.94 for the maximal value of . Finally, the maximal conversion fidelity that can be currently achieved in our system is given by the available SNR as: F QFCD ≤(SNR+1)/(SNR+2)=0.95 (see Supplementary Note 4 ). Note that the maximal fidelities can be achieved only if the conversion process preserves quantum coherence, which has been shown in various experiments both for qubit superposition [30] , [31] , [40] and entanglement [27] , [34] , [36] , [43] . We stress that the values for the various fidelities are given here only to infer the potential of our device in view of future qubit experiments. The correlation functions can also be used to infer the single photon nature of the heralded photon via the anticorrelation parameter α (ref. 44 ), where α =1 for coherent states and α =0 for perfect single photons. It has been shown that α can be estimated as (ref. 45 ). For the maximal measured value of , this would lead to α ≈0.2. Note that, with the current efficiencies of our SPDs at telecom wavelengths (0.1), a direct measurement of α for this high value of would require extremely long measurement times (several days) and has therefore not been performed. To use our QFCD for quantum networking applications, it should be demonstrated with long storage times. Long-lived Rb-based QMs have been demonstrated [14] , [46] , with storage time up to 100 ms (ref. 12 ). Our QFCD could be used with these more advanced QMs, as long as the retrieval efficiency is not affected (see for example, ref. 14 for a demonstration of an efficient and long lived QM). Our QFCD could be directly useful for some efficient quantum repeater architectures using DLCZ type QMs, where entanglement between remote quantum nodes is achieved by entanglement swapping involving the anti-Stokes photons [47] . In that case, the anti-Stokes photons are sent over long distances and must therefore be converted to telecom wavelengths. For protocols where entanglement between remote atomic ensembles is achieved by detection of the Stokes photon, such as the original DLCZ protocol [24] , or to achieve entanglement between a telecom photon and a stored spin excitation, the Stokes photon should then be converted. This would, however, require a significant increase of the SNR compared with our present experiment, since the Stokes emission probability has to be low to enable highly non-classical correlations. This may be achieved by using narrower filtering since the current value of 2.5 GHz is about two order of magnitude larger than the photon bandwidth. Obtaining higher SNR would be also interesting in view of using this interface in combination with single atom QMs emitting photons with duration of a few hundred nanoseconds [3] . In summary, we have demonstrated QFC to telecommunication wavelength of single photons emitted by a quantum memory, using a solid state integrated device. These results open the road to the use of integrated optics as a practical and flexible interface capable of connecting QMs to the optical fibre network. The wavelength flexibility offered by nonlinear crystals opens the door to QFC with other kind of QMs, such as solid state QMs [15] , [16] , [17] , [18] or single ions [4] , [6] , [7] . Our work is a step to extend quantum information networks to long distances and opens prospects for the coupling of different types of remote QMs via the optical fibre network. Quantum memory Our QM is based on an ensemble of 87 Rb atoms, trapped and cooled in a MOT. We use the D2 line at 780 nm, with the relevant states being | g ›=|5 2 S 1/2 , F =1›, | e ›=|5 2 P 3/2 , F ′=2› and | s ›=|5 2 S 1/2 , F =2›. The optical depth (OD) of the sample is measured to be ~12, when probing the | g › to | e › transition. At the beginning of the experimental sequence, the MOT is turned off and the atoms are optically pumped during 300 μs into the ground state | g ›. The write-read sequence is then repeated every 1.4 μs for 1,000 trials, before turning on the MOT again for 20 ms. About 46 MOTs per second are used, leading to a total trial number of ~46,000 per second. Several stages of filtering are used to isolate the Stokes and anti-Stokes fields from the write and read pulses, including spatial and polarization filters. After being coupled in a single mode fibre (efficiency 0.7), the Stokes field is also filtered spectrally using a monolithic Fabry-Perot cavity with linewidth ~60 MHz and transmission 0.20 (fibre to fibre). The total optical transmission experienced by the Stokes photon from the QM to the detector is 0.14 and the Stokes detection efficiency is 0.43. Quantum frequency converter device The crystal used for the QFCD is a 3 cm long PPLN-MgO waveguide. The pump light is at a wavelength of 1,569 nm and is generated by an extended cavity diode laser amplified by an erbium doped fibre amplifier. The measured coupling efficiencies into the waveguide are 68 and 60% for the pump and input modes, respectively. The input lens has a transmission of ~66% at 1,569 nm. The specified waveguide transmissions are about 78 and 62% at the pump and input wavelengths, respectively. At the waveguide output, two bandpass filters with a FWHM of 7 nm isolate the converted signal from the residual pump light. Each filter has a transmission of 93% at 1,552 nm, while it displays an OD of ~12 at 1,569 nm. A fibre Bragg grating with a linewidth of 2.5 GHz is also used to filter out the broadband noise generated by the pump beam. This allows us to reach a noise level of 1.42(6) × 10 −6 mW −1 ns −1 . Expected second order cross-correlation function The anti-Stokes detection probability after conversion can be expressed as , where p n is the probability to detect a noise photon. The quantity η tot = η dev · η trans · ( η d,1552 / η d,780 ) accounts for the QFCD efficiency ( η dev ), the passive losses between the anti-Stokes fibre output and the QFCD input ( η trans ~0.77) and the difference between the efficiencies of the SPDs used for 780 nm ( η d,780 =0.43) and 1,552 nm ( η d,1552 =0.1). The probability to detect an accidental coincidence between the Stokes and converted anti-Stokes fields is defined as p as c · p s and it is therefore given by η tot · p s · p as + p n · p s . In contrast, the coincidence probability will be given by η tot · p s,as + p n · p s . The factor η tot is the same as for p as , while the quantity p n · p s can be regarded as the probability to detect a noise photon conditioned on a previous detection of a Stokes photon (conditional noise). Using the definition of the second order cross-correlation function we obtain: We define the SNR as SNR= η tot · p s,as /( p n · p s ), which can be interpreted as the SNR for the detection of an anti-Stokes photon conditioned on a previous detection of a Stokes photon. With this definition, equation (2) can be cast in the form of equation (1). This formula presents a few remarkable aspects. In the limit of →+ ∞ (as it happens for p s → 0), equation (1) saturates to 1 + SNR. The SNR therefore expresses the maximum cross-correlation level achievable after conversion. In contrast, for high Stokes detection probabilities the function decreases. If we assume that SNR 1, then equation (1) gives . As it is detailed in Supplementary Note 3 , the SNR depends linearly on the probability to have a photon at the input of the QFCD. When we convert heralded single photons from the QM, this probability is given by the retrieval efficiency . Since is constant over a wide range of p s (see Fig. 2 ), for a fixed pump power the SNR can also be taken as constant in the same p s range. This assumption does not hold for high p s values. However, as we discussed above, in this case equation (1) does not depend on the SNR. Therefore, the SNR can be assumed as constant. How to cite this article: Albrecht, B. et al. A waveguide frequency converter connecting rubidium-based quantum memories to the telecom C-band. Nat. Commun. 5:3376 doi: 10.1038/ncomms4376 (2014).